Magnetically ultraresponsive nanoscavengers for next-generation water purification systems The development of sustainable, robust and energy efficient water purification technology is still challenging. Although use of nanoparticles is promising, methods are needed for their efficient recovery post treatment. Here we address this issue by fabrication of magnetically ultraresponsive ‘nanoscavengers’, nanoparticles containing synthetic antiferromagnetic core layers and functional capping layers. When dispersed in water, the nanoscavengers efficiently interact with contaminants to remove them from the water. They are then quickly collected (<5 min) with a permanent magnet, owing to their magnetically ultraresponsive core layers. Specifically, we demonstrate fabrication and deployment of Ag-capped nanoscavengers for disinfection followed by application of an external magnetic field for separation. We also develop and validate a collision-based model for pathogen inactivation, and propose a cyclical water purification scheme in which nanoscavengers are recovered and recycled for contaminant removal. Despite major efforts to develop water purification technology that is sustainable, robust and energy efficient, many human populations still lack access to clean and safe fresh water, especially in developing countries [1] , [2] . The major challenges are disinfection [3] , removal of chemical contaminants [4] , [5] and desalination [6] . Membrane filtration methods are well developed [7] , [8] , [9] , but fouling and high-energy consumption remain a major obstacle [10] , [11] . Although use of nanoparticles is promising [12] , [13] , [14] , [15] , methods are needed for their efficient recovery post treatment. In one way, particles can be mounted to a matrix [3] , [16] . However, this method blocks access to part of the particle surface and stops particle mobility and dispersal. Efficiency is compromised. An alternative is to create nanoparticles with a magnetic core—magnetically responsive nanoscavengers that can be deployed and recovered in a controlled manner. There are currently few methods of fabricating practical nanoscavengers with large magnetic cores and functional capping layers [4] , [17] , [18] . In this work, we advance fabrication technology with two contributions. First, we establish a technique for anchoring of inorganic nanoparticles to magnetic cores. Second, we fabricate a magnetic core, which is highly responsive to magnetic fields enabling collection of nanoscavengers with a permanent magnet. Magnetically ultraresponsive nanoscavengers were fabricated, which contain synthetic antiferromagnetic (SAF) core layers and functional capping layers. When dispersed in water, the nanoscavengers efficiently interact with contaminants to remove them from the water. They are then quickly collected (<5 min) with a permanent magnet, owing to their magnetically ultraresponsive core layers. Specifically, we demonstrate fabrication and deployment of Ag-capped nanoscavengers for disinfection followed by application of an external magnetic field for separation. We also develop and validate a collision-based model for pathogen inactivation, and propose a cyclical water purification scheme in which nanoscavengers are recovered and recycled for contaminant removal. Water purification system using nanoscavengers As shown in Fig. 1 , the water purification system is a two-step process. In Step 1, the nanoscavengers are dispersed in water containing micropollutants, such as pathogens, organic compounds and heavy metals. Both nanoscavengers and micropollutants move randomly due to Brownian motion, maximizing likelihood of collision. When this occurs, the active surface layer of the nanoscavenger can interact with the micropollutant, resulting in its absorption or detoxification/destruction. In Step 2, an external magnetic field is applied. The nanoscavengers are separated and collected, and purified water is discharged. This operational mode enables several advantages, including high-reaction efficiency, zero-energy input for the separation step and reuse of nanoscavengers. 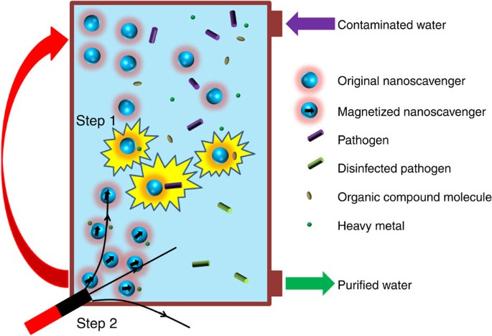Figure 1: Schematic representation of new water purification process. In Step 1, contaminated water is mixed with magnetic-core-anchored nanoscavengers. Treatment occurs when micropollutants in the water collide with nanoscavengers. Treatment of micropollutants, such as pathogens, organic compounds and heavy metals depends upon the materials used to cap the particles, which may enable disinfection, photo-catalytic degradation and adsorption. In Step 2, a magnetic separation process is applied to separate the nanoscavengers from purified water. The recovered nanoscavengers can then be reused in another cycle of water treatment. Figure 1: Schematic representation of new water purification process. In Step 1, contaminated water is mixed with magnetic-core-anchored nanoscavengers. Treatment occurs when micropollutants in the water collide with nanoscavengers. Treatment of micropollutants, such as pathogens, organic compounds and heavy metals depends upon the materials used to cap the particles, which may enable disinfection, photo-catalytic degradation and adsorption. In Step 2, a magnetic separation process is applied to separate the nanoscavengers from purified water. The recovered nanoscavengers can then be reused in another cycle of water treatment. Full size image Ag-SAF nanoscavengers for water disinfection Disk-shaped, multilayered SAF nanoparticles were fabricated with a well-established nanoimprint process [19] , [20] . Here to further fabricate nanoscavengers, we cover their surfaces with two functional capping layers (inset of Fig. 2a ), which remove targeted micropollutants from water. In one example, Ag-SAF nanoscavengers were fabricated for water disinfection by capping the SAF core with Ag, to make use of the well-known antibacterial effects of Ag ( [12] , [13] ). The Methods section describes the detailed fabrication process of Ag-SAF nanoscavengers. These particles have polycrystalline multilayers with the following layer sequence: Ag 20 nm, Ti 5 nm, Fe 5 nm, Ti 3 nm, Fe 5 nm, Ti 5 nm and Ag 20 nm ( Fig. 2a and Supplementary Fig. S1 ). 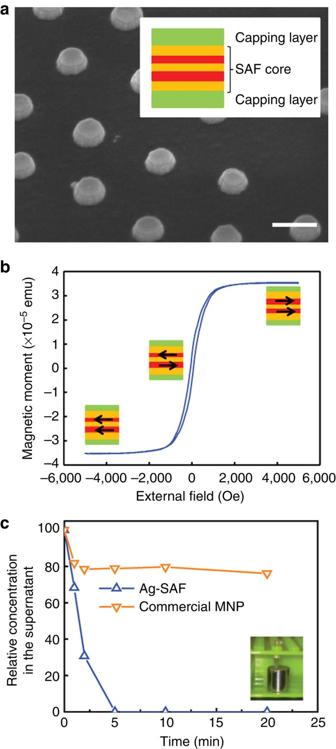Figure 2: Multilayered nanoscavengers and their magnetic response. (a) SEM image of Ag-SAF nanoscavengers immediately after fabrication, with a 200-nm scale for comparison. The inset shows the multilayer structure of the Ag-SAF nanoscavengers (SAF core covered by two Ag-capping layers). (b) Hysteresis loop measurement of these nanoscavengers. (c) Magnetic separation experiment, showing the relative concentration change in the supernatant with separation time. Inset figure is the experimental setup, where the centrifuge tube containing different MNP solution is placed on top of a permanent magnet for a set time period. The blue curve shows the behaviour of Ag-SAF nanoscavengers; the orange curve shows the behaviour of conventional commercial MNPs. Figure 2b is the hysteresis loop measurement of these nanoscavengers. Ideally, in the absence of a magnetic field, the moments of the two Fe layers are anti-parallel, leading to zero total moment. Remanence from fabrication defects is too small to cause aggregation of the nanoscavengers in water. Under a sufficiently high magnetic field, a parallel magnetic moment state is reached, and the total moment is saturated. From Fig. 2a , Ag-SAF nanoscavengers are around 150 nm in diameter, much larger than conventional superparamagnetic nanoparticles [21] . This results in a much higher single-particle magnetic moment. To demonstrate this advantage, Ag-SAF nanoscavengers were dispersed in water, collected in a centrifuge tube and placed above a permanent magnet (inset of Fig. 2c and Methods section). With no further optimization of the magnetic separation, over 99% of the originally dispersed nanoscavengers were collected within 5 min. When conventional commercial superparamagnetic iron-oxide magnetic nanoparticles (commercial MNPs) were tested under the same conditions, the concentration of nanoparticles in suspension barely changed after an initial drop of ~20% ( Fig. 2c ). This difference must be attributed to a difference in magnetic properties, rather than gravity, as both particle suspensions are stable in water for hours in the absence of a magnetic field. This result is consistent with previous observations, suggesting that SAF nanoparticles are readily manipulated with a permanent magnet [22] . These properties enable a simple separation. Figure 2: Multilayered nanoscavengers and their magnetic response. ( a ) SEM image of Ag-SAF nanoscavengers immediately after fabrication, with a 200-nm scale for comparison. The inset shows the multilayer structure of the Ag-SAF nanoscavengers (SAF core covered by two Ag-capping layers). ( b ) Hysteresis loop measurement of these nanoscavengers. ( c ) Magnetic separation experiment, showing the relative concentration change in the supernatant with separation time. Inset figure is the experimental setup, where the centrifuge tube containing different MNP solution is placed on top of a permanent magnet for a set time period. The blue curve shows the behaviour of Ag-SAF nanoscavengers; the orange curve shows the behaviour of conventional commercial MNPs. Full size image A disinfection test was performed with suspensions of either Gram-positive bacteria ( Enterococcus hirae ) or Gram-negative bacteria ( Escherichia coli ). Ag-SAF nanoscavengers were added, incubated and magnetically separated ( Fig. 3a and Methods section). The water was then assayed for bacteria. The effect of nanoscavenger addition depended upon incubation time and nanoscavenger dosage. Logarithmic removal rate (LRR) increased with incubation time, but with decreasing slope ( Fig. 3b ). The Ag-SAF nanoscavengers were more toxic to E. coli than to E. hirae as indicated by the much higher LRR at the same incubation time. This is expected, as the membrane of Gram-positive bacteria ( E. hirae ) contains a much thicker peptidoglycan layer than that of Gram-negative bacteria ( E. coli ), affording much better protection to Gram-positive bacteria. The LRR was proportional to the dosage of the Ag-SAF nanoscavengers ( Fig. 3c ). For E. coli , Ag-SAF nanoscavenger addition killed 99.9% at a dosage of 17 p.p.m. (as Ag) in 20 min. 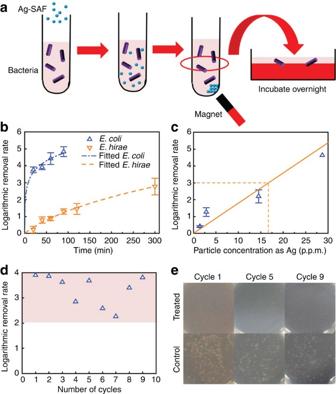Figure 3: Antibacterial effect of nanoscavengers. (a) Schematic representation of the experimental process: nanoscavenger addition, incubation, magnetic separation and analysis of the water sample. (b) LRR for bothE. coli(blue triangular dots) andE. hirae(orange inverted triangular dots) over time for a nanoscavenger dosage of 15.5 p.p.m. as Ag. The best fit for a collision model (blue dot-dashed line forE. coliand orange-dashed line forE. hirae) is shown. (c) Plot of LRR in response to different nanoscavenger dosages as Ag forE. coli. The blue triangular dots represent experimental data, and the solid orange line is the fitted curve. The dashed lines indicate that a nanoscavenger dosage of 17 p.p.m. can reach an LRR of 3. In bothbandc, the error bar at each data point reflects the s.d. of three repeated measurements of LRR. (d,e) Cyclic disinfection performance of the nanoscavengers. (d) The LRR ofE. coliin each cycle. (e) TypicalE. coliculturing results of a small portion of the treated water in cycle 1, 5 and 9. The first row is the treated sample with nanoscavengers, and the second row is the control without nanoscavengers. Figure 3: Antibacterial effect of nanoscavengers. ( a ) Schematic representation of the experimental process: nanoscavenger addition, incubation, magnetic separation and analysis of the water sample. ( b ) LRR for both E. coli (blue triangular dots) and E. hirae (orange inverted triangular dots) over time for a nanoscavenger dosage of 15.5 p.p.m. as Ag. The best fit for a collision model (blue dot-dashed line for E. coli and orange-dashed line for E. hirae ) is shown. ( c ) Plot of LRR in response to different nanoscavenger dosages as Ag for E. coli . The blue triangular dots represent experimental data, and the solid orange line is the fitted curve. The dashed lines indicate that a nanoscavenger dosage of 17 p.p.m. can reach an LRR of 3. In both b and c , the error bar at each data point reflects the s.d. of three repeated measurements of LRR. ( d , e ) Cyclic disinfection performance of the nanoscavengers. ( d ) The LRR of E. coli in each cycle. ( e ) Typical E. coli culturing results of a small portion of the treated water in cycle 1, 5 and 9. The first row is the treated sample with nanoscavengers, and the second row is the control without nanoscavengers. Full size image The cyclic disinfection performance of the Ag-SAF nanoscavengers was further investigated with E. coli . Figure 3d shows the LRR in different cycles. Though scattered, the LRR is typically within the range of 2 and 4 for up to nine cycles. The images of the cultured agar plates were also taken for cycle 1, 5 and 9 ( Fig. 3e ), showing essentially no bacterial growth for treated samples and extensive growth for untreated controls. A three-log reduction holds promise for practical applications because unlike conventional disinfectants, such as chlorine, the Ag-SAF nanoscavengers can be recovered and recycled to disinfect new batches of contaminated water. Mechanism for water disinfection using Ag-SAF nanoscavengers After separation, samples of supernatant and precipitate were further characterized. Only nanoscavengers were detected in the precipitate samples ( Fig. 4a ), and E. coli cells were only detected in the treated water ( Fig. 4b and Supplementary Fig. S2 ). This observation indicated that the decrease in E. coli in suspension was due to inactivation not attachment to nanoscavengers. A control experiment with Si-capped SAF nanoparticles had no antibacterial effect ( Supplementary Fig. S3 ), indicating that Ag chemistry has a role in disinfection. Many papers have evaluated the disinfection mechanism of Ag nanoparticles. Some have reported physical interactions between nanoparticles and bacteria, where particles attach to or penetrate the cell membrane [13] , [23] , [24] . In our experiments, such interaction was not involved. Ag-SAF nanoscavengers did not embed in the bacteria. Others have reported that dissolved Ag ions were the active agents of disinfection [25] , [26] , [27] , [28] . Here the concentration of dissolved Ag + in treated water was <10 p.p.b., below the reported threshold for disinfection [25] , but analyses of treated samples revealed trace levels of Ag inside inactivated E. coli cells ( Supplementary Fig. S4 ), indicating uptake of Ag from the Ag layers on the nanoscavengers. 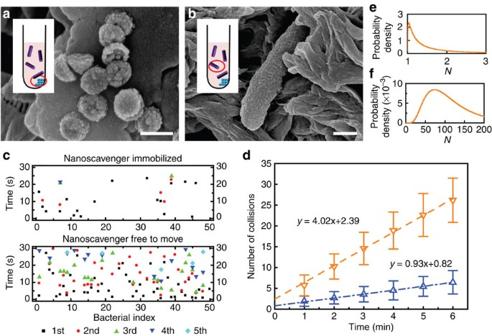Figure 4: Collision-based disinfection hypothesis. (a,b) SEM images of solution samples filtered through a fibre after water treatment. (a) Sediment solution, as demonstrated in the inset ofa. Scale bar, 200 nm. (b) Solution taken in the supernatant, as demonstrated in the inset ofb. Scale bar, 500 nm. (c) Recorded times of collision for 50 individual bacteria within 30 s obtained by Monte Carlo simulation, with nanoscavengers either immobilized or free to move. Different dot types indicate different number of times. (d) Average cumulative number of collisions for the case where nanoscavengers are either immobilized (blue triangular dots) or free to move (orange inverted triangular dots). Linear curves show model fit and collision frequencies of 0.93 min−1for a nanoscavenger that is immobile and 4.02 min−1for a nanoscavenger that is free to move. The error bars represent the s.d. of the number of collisions resulting from different simulation runs. (e,f) Distributions ofNfor (e)E. coliand (f)E. hirae. Figure 4: Collision-based disinfection hypothesis. ( a , b ) SEM images of solution samples filtered through a fibre after water treatment. ( a ) Sediment solution, as demonstrated in the inset of a . Scale bar, 200 nm. ( b ) Solution taken in the supernatant, as demonstrated in the inset of b . Scale bar, 500 nm. ( c ) Recorded times of collision for 50 individual bacteria within 30 s obtained by Monte Carlo simulation, with nanoscavengers either immobilized or free to move. Different dot types indicate different number of times. ( d ) Average cumulative number of collisions for the case where nanoscavengers are either immobilized (blue triangular dots) or free to move (orange inverted triangular dots). Linear curves show model fit and collision frequencies of 0.93 min −1 for a nanoscavenger that is immobile and 4.02 min −1 for a nanoscavenger that is free to move. The error bars represent the s.d. of the number of collisions resulting from different simulation runs. ( e , f ) Distributions of N for ( e ) E. coli and ( f ) E. hirae . Full size image Based on the above data, we developed a collision-based mechanism to describe the interaction between Ag-SAF nanoscavengers and bacteria. Both Ag-SAF nanoscavengers and bacteria undergo Brownian motion in water, and collisions ensue. When this happens, Ag is taken up by the bacteria, culminating in their death. The mechanisms of Ag toxicity are well documented: it can condense DNA molecules, react with thiol groups [29] and interact with enzymes of the respiratory chain [30] . Because Brownian motion is size dependent, the diffusion constant for nanoscavengers is much greater than that of bacteria, and nanoscavenger motion controls the frequency of collision. To confirm this intuition, we conducted a Monte Carlo simulation of the expected collisions between Ag-SAF nanoscavengers and bacteria ( Supplementary Note 1 and Supplementary Fig. S5 ). Fifty cells were simulated for two scenarios, assuming that either nanoscavengers have unconstrained motion or nanoscavengers are immobilized. The latter case has practical meaning, because it simulates the situation in which Ag nanoparticles are tightly bound to a matrix. Interestingly, within 30 s, two or three collisions have already occurred in the first case, whereas in the second case, most of the bacteria experience not more than one collision ( Fig. 4c ). A plot of the average cumulative number of collisions over time indicated a collision frequency of 4.02 min −1 for the first case and 0.93 min −1 for the second ( Fig. 4d ). Nanoscavenger mobility led to an immediate quadrupling of collision frequency. A death probability of 1/ N was defined as the probability of cell death upon collision with a nanoscavenger. Different species have different susceptibility to Ag as do different cells within the same species at different phases of their life cycle. In recognition of this fact, a log-normal distribution of N ranging from 1 to infinity was assigned to both E. coli and E. hirae ( Supplementary Note 2 ). The resulting expression was fit to experimental results ( Fig. 3b ). For E. coli , the distribution of N had an expected value of 1.29 and s.d. of 4.24; for E. hirae , the expected value was 115.9 and the s.d. was 70.2 ( Fig. 4e ). These results indicate that a single collision is sufficient to kill 78% of E. coli but only 0.9% of E. hirae . Our collision frequency model captured the salient features of the LRR in response to incubation time ( Fig. 3b ), and because collision frequency is proportional to nanoscavenger dosage, it also explains the increase in LRR with nanoscavenger dosage ( Fig. 3c ). In this paper, magnetically ultraresponsive nanoscavengers are fabricated, deployed for water purification, recycled and their mode of action modelled. These features suggest promise as a next-generation water treatment technology, particularly for point-of-use applications. Ag-capped nanoscavengers were developed as a model system for proof-of-concept, and these nanoscavengers were effective over several repeated cycles of disinfection. The bactericidal effect was adequately explained with a collision-based model. The average concentration of Ag inside inactivated bacteria is estimated to be <1% (based on Supplementary Fig. S4b ). Therefore, based on mass-balance calculation, at the dosage level of 14 p.p.m., Ag-SAF nanoscavengers can be repeatedly used for >4.5 × 10 5 times in treating water systems with 10 5 per ml bacteria as Ag. This value is inversely proportional to the concentration of bacteria and thus it may vary for real natural water system, which often contains different amount of bacteria. Admittedly, although these nanoscavengers work quite well in relatively clean systems, additional studies must be done in the future to examine their applicability towards messier systems that will contain not only microbes that need to be inactivated but also other materials that could react with and/or foul these particles. We note that the deployment, recovery and reuse of nanoscavengers is not limited to applications involving disinfection. By sequential deposition, different inorganic materials (metal, oxides and so on) can be capped to SAF nanoparticles. For instance, TiO 2 -capped SAF nanoparticles have also been fabricated ( Supplementary Fig. S6 ). These new particles have very promising application in water purification, as the capping layer itself has already been demonstrated to treat organic compound or heavy metal ions in water [14] , [15] . All the techniques involved (spin coating, nanoimprinting, etching, deposition, lift off and so on) are very well developed in industry, and minimal amount of labour is involved if these nanoscavengers are fabricated in an industry scale. Therefore, once a roll-to-roll-based process flow [31] is industrialized, these nanoscavengers can be fabricated with high efficiency and low cost. We also notice that other candidates, such as big-sized superparamagnetic nanoparticles (polycrystalline nanoparticles with diameter >100 nm), are also eligible as nanoscavengers [17] , [18] , [32] . In fact, those nanoparticles and SAF nanoparticles can be put together to tackle different micropollutants, given that they are coated with different capping layers with distinct functions. A collection of nanoscavengers could potentially enable parallel ‘one-pot’ treatment of diverse contaminants and contaminant mixtures. Fabrication and characterization of Ag-SAF nanoscavengers The detailed synthesis procedure is demonstrated in Supplementary Fig. S7 . Step 1: after the substrate (usually Si wafer) was cleaned by ultraviolet irradiation, it was spin coated by Durimide (Fujifilm Inc.; 3,000 r.p.m., post bake at 300 °C), polymethylglutarimide (PMGI SF3; MicroChem; 3,000 r.p.m., post bake at 200 °C) and poly (methyl methacrylate) (PMMA 75k200; Micro Resist Technology; 6,000 r.p.m., post bake at 140 °C). Step 2: a stamp with pillar structure (~150 nm in diameter, 390 nm pitch size) was nanoimprinted to make hole pattern in PMMA layer (180 °C, 40 bar and 60 s). Step 3: the wafer was dry etched with O 2 (100 mTorr, 20 s.c.c.m. and ~15 s) to remove the residue PMMA layer, followed by wet etching using the developer (MF26A; Shipley, 15 s) to form the undercut structure. Step 4: inorganic materials were deposited layer-by-layer onto the wafer to form the nanoscavengers in the holes and the residue sheet above PMMA layer. Step 5: lift-off process with acetone to dissolve PMMA layer and MF26A to dissolve PMGI layer; now the residue sheet had already peeled off and only nanoscavengers stayed above Durimide layer. Step 6: Durimide layer was removed by S-1165 (MicroChem Microposit), and nanoscavengers were released from the substrate. After a few runs of washing steps, nanoscavengers could be transferred to deionized water solution. Before particles were released from the substrate, a sample was taken for morphological characterization by secondary electron microscopy (SEM, FEI XL30; Sirion), and magnetic property measurements were performed using alternating gradient magnetometry (MicroMag 2900; Princeton Measurements Corporation). Magnetic separation of Ag-SAF nanoscavengers Two hundred microliter samples of both Ag-SAF nanoscavenger water solution and commercial MNP water solution (SMG-20-0005; Ocean Nanotech) were collected in different centrifuge tubes. These tubes were then placed above a permanent magnet for different time periods, allowing a fraction of the particles precipitated to the area close to the magnet. One hundred seventy microliters of supernatant in each sample was then transferred to a new tube, leaving 30 μl of solution containing nanoparticle precipitates. The relative concentration of Ag-SAF nanoscavengers in the supernatant was measured by inductively coupled plasma-mass spectroscopy (ICP-MS; Thermo Scientific XSERIES 2), after dissolving nanoscavengers in concentrated nitric acid, diluted by ultrapure distilled water and assayed by ICP-MS to determine the concentration of Ag + in solution. The relative concentration of iron-oxide nanoparticles was measured by the absorbance of the solution at 670 nm after homogeneous dispersal of the particles in water. Disinfection experiment with Ag-SAF nanoscavengers E. coli (JM109; Promega) was incubated in Luria-Bertani (LB) broth at 30 °C overnight, and E. hirae (ATCC No. 10541) was incubated in LB broth at 36 °C overnight. Both species were washed by distilled water at least four times before the disinfection experiment. Different amount of Ag-SAF nanoscavengers were mixed with ~10 6 ml −1 bacteria and incubated for a predefined time period. Each sample was then placed above a permanent magnet for 10 min, and Ag-SAF nanoscavengers precipitated to the bottom of the tube. For measurements of disinfection efficiency as a function of time, nanoscavenger dosage was maintained at 15.5 p.p.m. as Ag. For measurements of disinfection efficacy as a function of nanoscavenger dosage, the incubation time was fixed at 20 min. A subsample of supernatant was then transferred to a LB agar plate for spread plate analysis. This is a standard assay in which the subsample is spread over the agar surface of the plate with a sterile glass bar. The plates were then incubated at 30 °C (for E. coli ) and 37 °C (for E. hirae ) for 24 h. Each bacterium replicated to form a white colony. The number of the colonies was counted to determine the concentration of living E. coli or E. hirae in each sample. The Ag-SAF nanoscavenger dosage was represented by the Ag concentration measured by ICP-MS. The efficacy of the disinfection process was characterized by the LRR, which was defined as LRR=−log( C t / C 0 ), where C t and C 0 are the live bacteria concentrations in treated and untreated solutions, respectively. Cyclic performance of Ag-SAF nanoscavengers Initially, 1 ml of solution containing 14 p.p.m. Ag-SAF nanoscavengers (as Ag) and ~10 5 E. coli was incubated for 20 min, followed by magnetic separation with a permanent magnet. Nine hundred microliters of supernatant were transferred to a new tube, leaving 100 μl of suspension containing the particle precipitate. Samples of supernatant were removed to assay live E. coli after treatment. For the 100-μl suspension, particles were suspended by ultrasound, followed by addition of fresh E. coli and distilled water to give a total of 1 ml of solution containing ~10 5 ml E. coli . This process was repeated for nine cycles of disinfection. The supernatant and precipitate solution were collected for SEM and transmission electron microscopy (TEM; FEI Tecnai G2 F20 X-TWIN TEM). The pretreatment process of the E. coli supernatant and precipitate solution for SEM was described elsewhere [33] . Briefly, it consists of several steps. First, supernatant or precipitate samples were primarily fixed overnight in the fixative containing 0.1 M sodium cacodylate buffer (pH 7.3), 2% glutaraldehyde and 4% paraformaldehyde at 4 °C, then washed with the same buffer for 5 min. Second, they were immobilized onto a membrane filter. Third, secondary fixation was performed in 1% osmium tetroxide at 4 °C for 1–2 h, followed by washing with Milli-Q water for 10 min. Fourth, the samples were dehydrated in increasing concentrations of ethanol solution (50, 70, 90 and 100%), and critical point dried in 100% ethanol with liquid CO 2 . Finally, the samples were sputter coated with 10 nm of gold. To prepare TEM sample, supernatant samples were mixed with fixative containing 0.1 M sodium cacodylate buffer (pH 7.3), 2% glutaraldehyde and 4% paraformaldehyde at 4 °C, and then washed with the same buffer for 5 min. Then, one drop of the solution was spread and dried on a carbon-film-coated grid for TEM characterization. How to cite this article: Zhang, M. et al . Magnetically ultraresponsive nanoscavengers for next-generation water purification systems. Nat. Commun. 4:1866 doi: 10.1038/ncomms2892 (2013).